Direct atomic-scale confirmation of three-phase storage mechanism in Li4Ti5O12anodes for room-temperature sodium-ion batteries Room-temperature sodium-ion batteries attract increasing attention for large-scale energy storage applications in renewable energy and smart grid. However, the development of suitable anode materials remains a challenging issue. Here we demonstrate that the spinel Li 4 Ti 5 O 12 , well-known as a ‘zero-strain’ anode for lithium-ion batteries, can also store sodium, displaying an average storage voltage of 0.91 V. With an appropriate binder, the Li 4 Ti 5 O 12 electrode delivers a reversible capacity of 155 mAh g −1 and presents the best cyclability among all reported oxide-based anode materials. Density functional theory calculations predict a three-phase separation mechanism, 2Li 4 Ti 5 O 12 +6Na + +6e − ↔Li 7 Ti 5 O 12 +Na 6 LiTi 5 O 12 , which has been confirmed through in situ synchrotron X-ray diffraction and advanced scanning transmission electron microscope imaging techniques. The three-phase separation reaction has never been seen in any insertion electrode materials for lithium- or sodium-ion batteries. Furthermore, interfacial structure is clearly resolved at an atomic scale in electrochemically sodiated Li 4 Ti 5 O 12 for the first time via the advanced electron microscopy. In the energy storage field, lithium-ion batteries have been investigated substantially in the past few decades and used widely in many aspects of our society [1] . However, one shall always be prepared for the exhaustion of lithium resource should lithium-ion battery-based electric vehicle technology be applied in large scale as expected in the near future [2] , [3] . As an alternative technology, room-temperature sodium-ion batteries, which were originally investigated in parallel with lithium-ion batteries, have again aroused interest recently for large-scale stationary energy storage in the applications of renewable energy and smart grid because of their low cost and the infinite sodium resources [2] , [4] , [5] , [6] , [7] . Recent investigations on sodium-ion batteries were mainly focused on the cathode materials, for example, Na x CoO 2 (refs 8 , 9 ), NaCrO 2 (refs 10 , 11 ), Na x MnO 2 (ref. 12 ), NaNi 0.5 Mn 0.5 O 2 (ref. 13 ), NaNi 1/3 Mn 1/3 Fe 1/3 O 2 (ref. 14 ), P2-type Na 2/3 [M x Mn 1− x ]O 2 (refs 15 , 16 ), Na 1.0 Li 0.2 Ni 0.25 Mn 0.75 O δ (ref. 17 ), Na 2 MPO 4 F (ref. 2 ), Na 3 V 2 (PO 4 ) 3 /C (refs 18 , 19 ), and so on. In contrast, very few anode materials were reported to be viable [5] , [20] . Among the limited number of anode materials [13] , [21] , [22] , [23] , [24] , [25] , [26] , [27] , [28] , [29] , hard carbon is the only candidate possessing both high storage capacity and good cycling [13] , [23] . However, as the sodium storage voltage in hard carbon is relatively low and near zero versus Na + /Na, this would result in sodium metal deposition on its surface in an improper operation or during fast charging, giving rise to major safety concern. The other interesting electrode material is Na 2 Ti 3 O 7 , but with a storage voltage at 0.2 V, the risk of sodium plating is the same; besides the material shows hysteresis and the cycling performance is not satisfied [24] . Therefore, it is desirable to develop other new anode materials with relatively high storage voltage. We have reported spinel Li 4 Ti 5 O 12 , which is well known as a ‘zero-strain’ anode material for long-life stationary lithium-ion batteries [30] , [31] , as anode material for room-temperature sodium-ion battery [32] . These preliminary results show an average storage voltage at ca. 0.9 V and a reversible capacity of 145 mAh g −1 . Compared with hard carbon, Li 4 Ti 5 O 12 sacrifices the energy density to some extent, but the relatively high storage voltage versus sodium metal makes it intrinsically much safer than hard carbon. As can be seen from the ex situ X-ray diffraction (XRD) result in our previous report [32] , several new peaks corresponding to the peaks of Li 4 Ti 5 O 12 but with lower diffraction angles appear during the sodium insertion process; by a rough calculation we found that a new cubic structure with larger lattice parameters (ca. 13% volume expansion compared with Li 4 Ti 5 O 12 ) is formed. Herein, we further show that Li 4 Ti 5 O 12 can exhibit excellent sodium storage performance in an optimized condition for sodium-ion batteries. By using appropriate binders, the Li 4 Ti 5 O 12 electrode displays the best cyclability among the existing oxide-based anode material for sodium-ion batteries. It shows a stable specific capacity of 155 mAh g −1 with coulombic efficiency >99%. With the help of density functional theory (DFT) calculations, we predict a three-phase separation mechanism. Then the three-phase separation reaction is confirmed via in situ synchrotron XRD measurement and advanced scanning transmission electron microscope (STEM) imaging techniques. To the best of our knowledge, this is the first time that a three-phase reaction has been found among the insertion electrodes for Li-/Na-ion batteries. Moreover, the interfacial structure among three phases with sharp phase boundaries is clearly resolved at atomic scale in the electrochemically sodiated Li 4 Ti 5 O 12 . Sodium storage performance To overcome the capacity fading resulting from volume expansion of insertion material, we tried to optimize the composite electrode by using high tensile-strength binders, sodium alginate (NaAlg) or carboxymethyl-cellulose sodium (Na-CMC), both of which were used to improve the cyclic performance of the Li-ion battery electrode materials with large volume expansion, for example, nano-Si anode [33] , [34] . An advantage for future green processing, these polymers are water soluble. 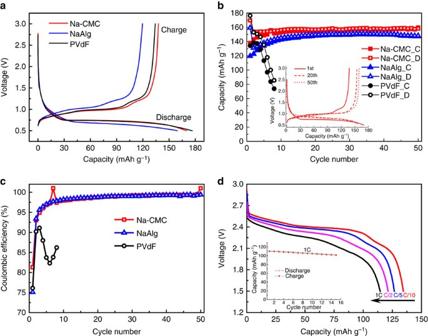Figure 1: Electrochemical performance of Li4Ti5O12in sodium-ion batteries. The Li4Ti5O12electrode was cycled in NaFSI/EC:DEC electrolyte at a current rate of C/10. (a) Comparison of the initial discharge/charge curves of PVdF, NaAlg and Na-CMC electrodes. (b) Cyclic performances of PVdF, NaAlg and Na-CMC electrodes (inset is the 1st, 10th, 50th discharge/charge profiles of Na-CMC electrode). (c) Coulombic efficiencies versus cycle number of PVdF, NaAlg and Na-CMC electrodes. (d) Discharge profiles of Li4Ti5O12//Na3V2(PO4)3/C sodium full cell at various rates (inset is the cyclic performance of the full cell at 1C rate). Figure 1a shows the initial discharge and charge curves of polyvinylidene difluoride (PVdF)-, NaAlg- and Na-CMC-based electrodes cycled in a novel NaFSI/EC:DEC electrolyte. The NaAlg electrode displays a relatively low discharge capacity (159 mAh g −1 ) and a coulombic efficiency of 75.1%, while the Na-CMC electrode exhibits a high discharge capacity of 170 mAh g −1 and a coulombic efficiency of 81.3%. The low coulombic efficiency could be attributed to the formation of a solid electrolyte interphase layer on the Li 4 Ti 5 O 12 nano-particles ( Supplementary Fig. S1 ). Figure 1b illustrates the cyclic performance and coulombic efficiencies of Li 4 Ti 5 O 12 electrodes with different binders. The capacity fades rapidly for the conventional PVdF electrode. In the case of NaAlg electrode, a low capacity is obtained after the first cycle; in the subsequent cycles, the reversible capacity increases and reaches a stable value of 148 mAh g −1 after 20 cycles. However, the Na-CMC electrode exhibits a stable capacity up to 155 mAh g −1 and a coulombic efficiency >99% as well as an excellent cyclic performance just after few cycles, thus validating Na-CMC as a better binder for Li 4 Ti 5 O 12 . Note that after optimization, Li 4 Ti 5 O 12 outperforms all existing oxide-based anode materials for sodium-ion batteries (see Table 1 ). Galvanostatic intermittent titration technique (GITT) studies on the Li 4 Ti 5 O 12 electrode confirm an average potential of 0.91 V for sodium storage ( Supplementary Fig. S2 ). Figure 1: Electrochemical performance of Li 4 Ti 5 O 12 in sodium-ion batteries. The Li 4 Ti 5 O 12 electrode was cycled in NaFSI/EC:DEC electrolyte at a current rate of C/10. ( a ) Comparison of the initial discharge/charge curves of PVdF, NaAlg and Na-CMC electrodes. ( b ) Cyclic performances of PVdF, NaAlg and Na-CMC electrodes (inset is the 1st, 10th, 50th discharge/charge profiles of Na-CMC electrode). ( c ) Coulombic efficiencies versus cycle number of PVdF, NaAlg and Na-CMC electrodes. ( d ) Discharge profiles of Li 4 Ti 5 O 12 //Na 3 V 2 (PO 4 ) 3 /C sodium full cell at various rates (inset is the cyclic performance of the full cell at 1C rate). Full size image Table 1 The sodium storage properties for different reported anode materials for sodium-ion batteries. Full size table The Li 4 Ti 5 O 12 as an anode in a full cell was also demonstrated using Na 3 V 2 (PO 4 ) 3 /C as cathode. Preliminary results show that the full cell gives rise to an average operating voltage plateau at ~2.4 V and appropriate rate and cyclic performance ( Fig. 1d ). The performance can be further enhanced by optimization of both electrodes and their weight ratio. DFT simulations DFT-based first-principles calculations were employed to understand the sodium insertion mechanism of Li 4 Ti 5 O 12 electrode. Spinel Li 4 Ti 5 O 12 (abbr. Li4) can be more precisely written as [Li 3 ] 8 a V 16 c [Ti 5 Li] 16 d O 12 (V: vacancy), wherein three Li + ions occupy the 8 a tetrahedral interstitial sites and the remaining one Li + and all Ti 4+ ions reside in the 16 d octahedral interstitial sites of cubic close-packed oxygen sublattice. Upon discharge in a Li-ion battery (half cell), three Li can be inserted into the 16 c sites accompanied by pushing three Li + ions from the 8 a sites to the 16 c sites [35] , [36] , leading to transformation from the Li4 phase to the V 8 a [Li 6 ] 16 c [Ti 5 Li] 16 d O 12 (abbr. Li7) phase. The reaction could be represented as: This is a typical two-phase reaction and delivers a flat voltage plateau of 1.55 V versus Li + /Li. The lattice volume difference between the Li4 and Li7 phases is negligibly small. With structure model shown in Fig. 2a , above features concerning the lithiation process could be well reproduced by the DFT calculations ( Supplementary Fig. S3 ). This agreement gives us confidence to investigate the subsequent sodium insertion process using the same method. 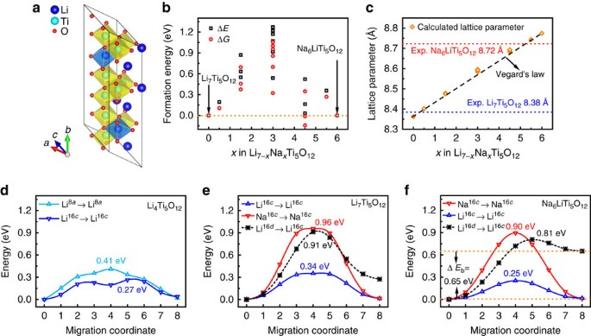Figure 2: DFT calculations. (a) Schematic illustration of the structure model adopted in structure optimization. Li16dO6and Ti16dO6octahedra are plotted in blue and yellow, respectively. (b) Calculated formation energyand Gibbs free energy (taking into account of the configurational entropies given a completely random Li/Na distribution at 16dsite,) of Li7−xNaxTi5O12, positive (negative) value indicates thermodynamically driven Na-Li segregation (mixing) at 16csites. (c) Optimized lattice parameters of Li7−xNaxTi5O12. Optimized hopping barriers of Li and Na ions in Li4Ti5O12(d), Li7Ti5O12(e) and Na6LiTi5O12(f). For Na6LiTi5O12,ΔEbis defined as. Figure 2: DFT calculations. ( a ) Schematic illustration of the structure model adopted in structure optimization. Li 16 d O 6 and Ti 16 d O 6 octahedra are plotted in blue and yellow, respectively. ( b ) Calculated formation energy and Gibbs free energy (taking into account of the configurational entropies given a completely random Li/Na distribution at 16 d site, ) of Li 7− x Na x Ti 5 O 12 , positive (negative) value indicates thermodynamically driven Na-Li segregation (mixing) at 16 c sites. ( c ) Optimized lattice parameters of Li 7− x Na x Ti 5 O 12 . Optimized hopping barriers of Li and Na ions in Li 4 Ti 5 O 12 ( d ), Li 7 Ti 5 O 12 ( e ) and Na 6 LiTi 5 O 12 ( f ). For Na 6 LiTi 5 O 12 , ΔE b is defined as . Full size image Inferring from the ex situ XRD results [32] , a new phase sharing the same cubic structure but with a larger lattice parameter emerges after the sodium insertion. Electrochemical measurements show that about three Na ions can be inserted into one formula unit of Li 4 Ti 5 O 12 , whereas elemental analysis of the electrolyte and the counter electrode indicates that no lithium is released after cycling. As Na + ion is too large to occupy the 8 a tetrahedral site, it is more likely to occupy the 16 c octahedral site after being inserted into Li4. Thus, the sodium insertion process is expected to be analogous to the lithium insertion process. Supposing Li at 16 d site is fixed during the electrochemical process, formation of V 8 a [Na x Li 6− x ] 16 c [Ti 5 Li] 16 d O 12 (0≤ x ≤6) is expected. To study the Li/Na distribution in 16 c octahedral site, the formation energy of V 8 a [Na x Li 6− x ] 16 c [Ti 5 Li] 16 d O 12 with respect to its two end members, V 8 a [Li 6 ] 16 c [Ti 5 Li] 16 d O 12 and V 8 a [Na 6 ] 16 c [Ti 5 Li] 16 d O 12 (abbr. Na6Li), are calculated. Results shown in Fig. 2b indicate that the Li/Na solid solution at 16c sites is not energetically favourable, which suggests a phase separation of Li7 and Na6Li. Conversely, if we hypothesize that the solid solution reaction dominates the discharge/charge process, the resulting XRD pattern will shift gradually at different discharge/charge states, as the computational results show that the lattice parameters of V 8 a [Na x Li 6− x ] 16 c [Ti 5 Li] 16 d O 12 (0≤ x ≤6) obey Vegard’s law ( Fig. 2c ). Actually, the diffraction peaks do not shift significantly from the ex situ XRD patterns, thus invalidating the solid solution reaction as a proper explanation for the sodium insertion process. Accordingly, we predict the following three-phase separation mechanism for the sodium insertion process (in a half cell): Above equation suggests that two new phases, that is, Na6Li and Li7, are created after the Na is inserted into the Li4 phase, which is consistent to the Rietveld refinement result of XRD pattern for the chemically sodiated Li 4 Ti 5 O 12 ( Supplementary Fig. S4 ). According to the three-phase separation mechanism, both the calculated storage voltage (0.88 V) and lattice volume expansion (13%) agree well with the experimental values (0.91 V and 12.5%, respectively). Kinetic properties of this reaction are assessed by evaluating the hopping barriers of both Li + and Na + ions ( Fig. 2d–f ), leading to the following results. (1) The aforementioned assumption that Li 16 d ions are nearly fixed in the lattice is confirmed here. In Li4 phase, the Li 16 d displaced from the 16 d site will restore the original position after relaxation and therefore not presented here; in Li7 phase, the hopping barrier of Li 16 d is much higher than that of Li 16 c , indicating a much lower migration probability; in Na6Li phase, even though the energy barrier of Li + migration from 16 d to a 16 c site is comparable to that of Na + migration, the reverse migration (Li 16 c →Li 16 d ) has a much lower barrier (by 0.65 eV) and thus its hopping possibility exceeds that of the Li 16 d →Li 16 c direction by ten orders of magnitude at room temperature, making the Li 16 d migration practically impossible. (2) Kinetics of Na + ion is much slower than that of Li + ion. As the hopping barrier of Li + ion is much lower than that of Na + ion, a much higher migration probability of the former is expected, viz. Li + ion will relax to their ground state following the movement of Na + ion instantaneously, as the latter diffuses much slower than the former. Three-phase separation mechanism On the basis of the above analysis, we may describe the sodium insertion/extraction process in a single Li 4 Ti 5 O 12 particle as follows: upon discharge, Na + ions will occupy 16 c sites exclusively to form Na6Li phase and at the same time, Li 8 a ions are pushed to the nearest neighbour Li4 phase forming Li7 phase, which is equivalent to a lithium insertion process. In this manner two new phases, Na6Li and Li7, are created ( Fig. 3a ). As the discharge continues, taking no account of new nucleation of Na6Li, sodium insertion will proceed on the Na6Li/Li7 boundary, resulting in the transformation of Li7 into Na6Li phase and thus pushing this boundary forward. Meanwhile, the Li 16 c ions from the initial Li7 phase will diffuse into the nearby Li4 phase to form Li7 phase, and thus the Li7/Li4 boundary proceeds. Ideally, all of the Li4 phase would be exhausted at the end of the discharge, leaving coexistence of Li7 and Na6Li phases with equivalent amount. In the charging process ( Fig. 3b ), Na + ions are extracted from the Na6Li/Li4 boundary leaving vacancies at both 8 a and 16 c sites, and then the Li ions, driven by the thermodynamic force, will fill the 8 a sites to form Li4 phase, until the end of charge. Compared with the conventional two-phase lithiation mechanism of Li 4 Ti 5 O 12 electrode ( Fig. 3c ), coexistence of three phases with two kinds of phase-boundaries features the sodium insertion/extraction process. 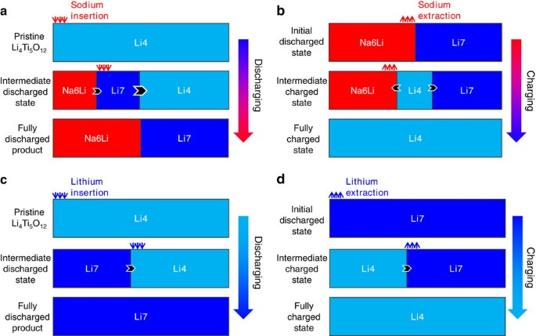Figure 3: Comparison between sodiation and lithiation processes in Li4Ti5O12. Discharging (a) and charging (b) processes in a sodium-ion battery. Discharging (c) and charging (d) processes in a lithium-ion battery. Li4Ti5O12(Li4), Li7Ti5O12(Li7) and Na6LiTi5O12(Na6Li) phases are represented by light blue, blue and red colours, respectively. Directions of phase boundary movement are marked by black arrows. Figure 3: Comparison between sodiation and lithiation processes in Li 4 Ti 5 O 12 . Discharging ( a ) and charging ( b ) processes in a sodium-ion battery. Discharging ( c ) and charging ( d ) processes in a lithium-ion battery. Li 4 Ti 5 O 12 (Li4), Li 7 Ti 5 O 12 (Li7) and Na 6 LiTi 5 O 12 (Na6Li) phases are represented by light blue, blue and red colours, respectively. Directions of phase boundary movement are marked by black arrows. Full size image Hypothesizing that the thermodynamic equilibrium could always be achieved during discharge/charge, the resulting voltage profile should be a plateau, which is a characteristic of the phase separation reaction. However, the plateau feature might be penalized by the slow reaction kinetics. This phenomenon could be seen in high rate discharge/charge in other phase separation materials, for example, LiFePO 4 (ref. 37 ). Through DFT simulations we have shown that the transport kinetics of Na + ion is slow in this system and, therefore, the actual reaction path might deviate from thermodynamic equilibrium state, resulting in the sloped discharge/charge curve. Actually, the equilibrium state is not achieved even after a relaxation time of 12 h in our GITT measurement ( Supplementary Fig. S2 ), further indicating that the electrochemical process of Li 4 Ti 5 O 12 electrode cycled in a Na-ion battery system is kinetically controlled. In situ synchrotron XRD The electrochemical sodium insertion/extraction process is also investigated via in situ synchrotron XRD. We can see from Fig. 4 that a new set of peaks corresponding to Na6Li phase appears upon discharge and disappears in the following charge process, which characterizes a phase separation reaction instead of solid solution reaction. However, the new phase delays regarding to the discharging process: diffraction peaks corresponding to the Na6Li phase do not appear till the end of the discharge, and its intensity reach a maximum during the subsequent charging process. Analogous phenomenon has also been reported in the LiFePO 4 cathode material for Li-ion batteries (refs 38 , 39 ). Under a phase separation mechanism, the insertion process is accompanied by the nucleation and growth of the new phases, while the XRD measurement as a diffraction technique can only probe the new phases larger than a certain domain size. Owing to the slow Na + ion kinetics, such a delay is not unexpected. 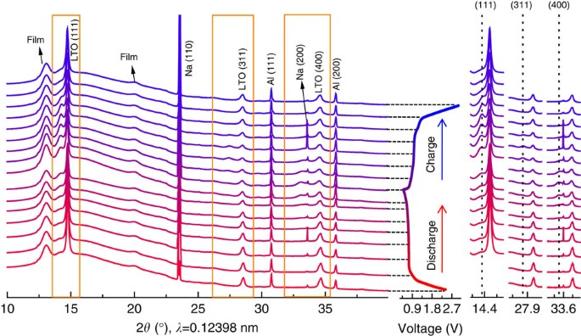Figure 4:In situsynchrotron XRD patterns. The data were recorded during the first cycle for the Li4Ti5O12electrode in a sodium-ion battery system. For the Li4/Li7 phases, the main peaks correspond to (111), (311) and (400) reflections. These regions are highlighted in the right column and peaks corresponding to the Na6Li phase are marked by black dotted lines. Figure 4: In situ synchrotron XRD patterns. The data were recorded during the first cycle for the Li 4 Ti 5 O 12 electrode in a sodium-ion battery system. For the Li4/Li7 phases, the main peaks correspond to (111), (311) and (400) reflections. These regions are highlighted in the right column and peaks corresponding to the Na6Li phase are marked by black dotted lines. Full size image Although the leading feature of the in situ synchrotron XRD patterns indicates a phase separation reaction, a slight peak shift suggests a solid solution reaction at the beginning of discharge. It is found that the peaks corresponding to Li4/Li7 phase shift towards lower angle region at discharge and then shift backward upon charging ( Supplementary Fig. S5 ). It has been reported that the representative phase-separation electrode materials for Li-ion batteries, for example, Li 4 Ti 5 O 12 (ref. 40 ) and LiFePO 4 (ref. 41 ), also have solid solution regions nearby the stoichiometric end members. The solid solution phase in three-phase reaction could be more complex than its counterpart in the two-phase reaction, as there is one more degree of freedom. In general, the solid solution could be written as Li 3+ α Na β [LiTi 5 ]O 12 (close to the Li4 phase), Li 6− α − β Na α V β [LiTi 5 ]O 12 (close to the Li7 phase), Na 6− α − β Li α V β [LiTi 5 ]O 12 (close to the Na6Li phase). Nonetheless, the solid solution is entropy driven and we do not think it is predominant at room temperature. STEM imaging To further confirm the three-phase sodium insertion mechanism, spherical aberration-corrected STEM [42] were employed to obtain a direct vision of the atomic structure. Recently, the STEM technique has been proved to be powerful in providing comprehensive information of electrode materials for Li-ion batteries at the atomic scale [43] . Within this technology, the contrast of the annular-bright-field (ABF) image exhibits a Z 1/3 dependency in contrast to the Z 1.7 dependency for high-angle annular-dark-field (HAADF) imaging, where Z represents the atomic number. Consequently, the light elements, for example, H and Li, which are almost indiscernible in the HAADF approach, can be indentified with the ABF method [44] . For Li 4 Ti 5 O 12 , [110] projection is most suitable for observation, because separated columns of Li, O and Ti ions (neglecting the randomly distributed Li 16 d ) are aligned in this direction ( Fig. 5a ). As Li 4 Ti 5 O 12 and Li 7 Ti 5 O 12 share an almost identical [Ti 5 Li] 16 d O 12 host, they are nearly indistinguishable in HAADF images because of no contrast of Li columns ( Fig. 5b ). However, in the ABF image, the Li contrasts can be identified in 8 a ( Fig. 5c ) and 16 c sites ( Fig. 5f ) for Li 4 Ti 5 O 12 and the Li 7 Ti 5 O 12 , respectively. The corresponding line profiles give a much clearer picture for the Li-ion position ( Fig. 5d ). 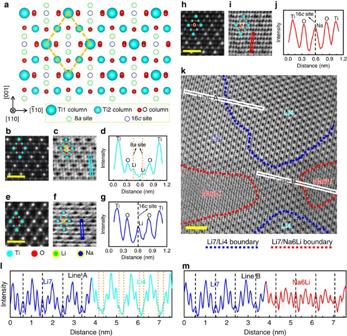Figure 5: STEM imaging of a three-phase coexistence region. (a) Crystal structure of spinel Li4Ti5O12viewed from the [110] crystallographic direction showing separated Ti and O columns. Ti1 and Ti2 columns with different atom densities are represented by balls of different size. HAADF (b), ABF (c) images and ABF line profile (d) of Li4Ti5O12(Li4) phase. Scale bar, 1 nm. HAADF (e), ABF (f) images and ABF line profile (g) of Li7Ti5O12(Li7) phase. Scale bar, 1 nm. HAADF (h), ABF (i) images and ABF line profile (j) of Na6LiTi5O12(Na6Li) phase. Scale bar, 1 nm. (k) ABF image in the half electrochemically sodiated Li4Ti5O12nano-particle. In ABF line profile, the contrast is inverted for a convenient visualization. Scale bar, 2 nm. (l,m) Line profiles crossing the Li7/Li4 (line A) and Li7/Na6Li (line B) boundaries, respectively. Figure 5: STEM imaging of a three-phase coexistence region. ( a ) Crystal structure of spinel Li 4 Ti 5 O 12 viewed from the [110] crystallographic direction showing separated Ti and O columns. Ti1 and Ti2 columns with different atom densities are represented by balls of different size. HAADF ( b ), ABF ( c ) images and ABF line profile ( d ) of Li 4 Ti 5 O 12 (Li4) phase. Scale bar, 1 nm. HAADF ( e ), ABF ( f ) images and ABF line profile ( g ) of Li 7 Ti 5 O 12 (Li7) phase. Scale bar, 1 nm. HAADF ( h ), ABF ( i ) images and ABF line profile ( j ) of Na 6 LiTi 5 O 12 (Na6Li) phase. Scale bar, 1 nm. ( k ) ABF image in the half electrochemically sodiated Li 4 Ti 5 O 12 nano-particle. In ABF line profile, the contrast is inverted for a convenient visualization. Scale bar, 2 nm. ( l , m ) Line profiles crossing the Li7/Li4 (line A) and Li7/Na6Li (line B) boundaries, respectively. Full size image In the HAADF images of the electrochemically sodiated Li 4 Ti 5 O 12 , a significant contrast is observed at 16 c site ( Fig. 5h ), which is distinguished from both Li4 and Li7 phases. That means atoms with large Z emerged at 16 c sites after the sodium insertion, and hence it is reasonably attributed to the formation of Na6Li phase. Above experimental observations agree well with the simulated STEM images ( Supplementary Fig. S6 ). In the ABF images of Na6Li phase ( Fig. 5i ), the contrast gap between different atomic columns is not so large as in Li7 and Li4 phases, as shown in the line profile ( Fig. 5j ). Accordingly, we find a three-phase coexistence region in the half-discharged sample ( Fig. 5k ), with distinguishable Li7/Li4 and Li7/Na6Li phase boundaries ( Fig. 5l ). Determining the interfacial structure is critical for understanding the ionic transport and movement of phase boundary in a typical phase transition reaction. To the best of our knowledge, little attention has been paid to the interfacial issues in atomic scale in a battery system. Very recently, we observed an ordered interface with staging structure between LiFePO 4 and FePO 4 phases in a partially chemically delithiated Nb-doped LiFePO 4 sample [45] . Here this is the first time to visualize clearly the interface at atomic scale for a phase transition reaction in an electrochemically inserted sample, which nearly reflects the real situation occurred in a battery. It can be seen that the two-phase boundaries of Li7/Li4 and Li7/Na6Li are sharp and dislocation free ( Fig. 5l ), which is consistent with our previous observation in a chemically lithiated Li 4 Ti 5 O 12 (ref. 46 ). In the fully discharged samples, coexistence of the two final phases Li7 and Na6Li are also identified with sharp phase boundary between them ( Fig. 6 ). These results agree well with our theoretical prediction and hence make strong evidence for the three-phase separation mechanism. Compared with the straight line in lithiated Li 4 Ti 5 O 12 , nevertheless, we note that the arrangement of the atomic columns is not that regular ( Supplementary Fig. S7 ). This could be ascribed to the coherency strain resulted from the lattice mismatch between Li4/Li7 and Na6Li phases. 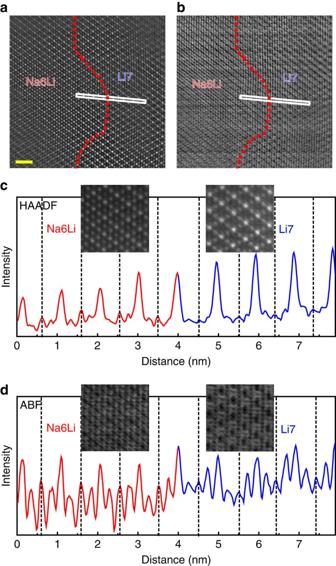Figure 6: STEM images of fully discharged Li4Ti5O12. HAADF (a) and ABF (b) images. Scale bar, 2 nm. Line profiles of HAADF (c) and ABF (d), where 16csites are labelled by black dash lines. In ABF line profile, the contrast is inverted for a convenient visualization. Figure 6: STEM images of fully discharged Li 4 Ti 5 O 12 . HAADF ( a ) and ABF ( b ) images. Scale bar, 2 nm. Line profiles of HAADF ( c ) and ABF ( d ), where 16 c sites are labelled by black dash lines. In ABF line profile, the contrast is inverted for a convenient visualization. Full size image In addition, we study the elemental distribution of the electrode material at the 5th cycle using energy-dispersive X-ray spectroscopy (EDX)-STEM mapping. As can be seen in Fig. 7a–d , both oxygen (red) and titanium (green) elements were distributed uniformly in the sodium-inserted Li 4 Ti 5 O 12 nano-particles. In contrast, the sodium element (yellow) was unevenly distributed. This is consistent with the three-phase separation scenario, according to which the Na-containing phase could occupy up to half of the whole particle at the end of discharge. The elemental distribution of the recharged particle is illustrated in Fig. 7e–h , from which we can see almost no signal of sodium element, indicating that the Na ions are fully extracted from the electrode after charging. 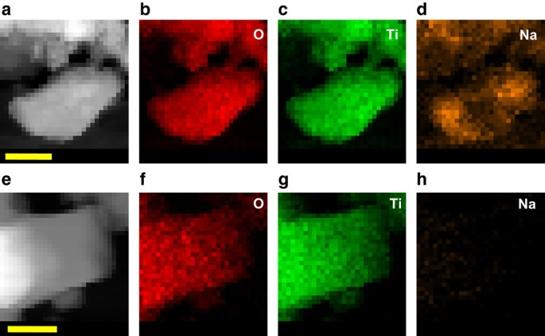Figure 7: EDX-STEM mapping of Li4Ti5O12nano-particles. (a) STEM image of a Li4Ti5O12nano-particle at the 5th discharged state;b,canddare the corresponding elemental mapping of the O, Ti and Na elements, respectively. Scale bar, 100 nm. (e) STEM image of a Li4Ti5O12nano-particle at the 5th charged state;f,gandhare the corresponding elemental mapping of the O, Ti and Na elements, respectively. Scale bar, 30 nm. Figure 7: EDX-STEM mapping of Li 4 Ti 5 O 12 nano-particles. ( a ) STEM image of a Li 4 Ti 5 O 12 nano-particle at the 5th discharged state; b , c and d are the corresponding elemental mapping of the O, Ti and Na elements, respectively. Scale bar, 100 nm. ( e ) STEM image of a Li 4 Ti 5 O 12 nano-particle at the 5th charged state; f , g and h are the corresponding elemental mapping of the O, Ti and Na elements, respectively. Scale bar, 30 nm. Full size image As already discussed above, by combining first-principles calculations with advanced spherical aberration-corrected STEM, we have confirmed a novel three-phase separation mechanism discussed here for sodium storage in Li 4 Ti 5 O 12 . With the insertion of Na into Li 4 Ti 5 O 12 , Na + ion will occupy the vacancy of 16 c site in Li 4 Ti 5 O 12 and simultaneously Li + ion at 8 a site will be, similar to Li insertion, driven into 16 c site due to the coulombic repulsion between occupied 8 a and 16 c sites, forming V 8 a [Li x Na 6− x ] 16 c [LiTi 5 ] 16 d O 12 . However, owing to the different size of Li + and Na + ions, V 8 a [Li x Na 6− x ] 16 c [LiTi 5 ] 16 d O 12 will separate into two rock-salt phases of V 8 a [Na 6 ] 16 c [LiTi 5 ] 16 d O 12 and well-known V 8 a [Li 6 ] 16 c [LiTi 5 ] 16 d O 12 . This three-phase reaction, where two guest ions ( viz. Li + and Na + ) of different size and mobility occupy the same crystallographic sites of [LiTi 5 ] 16 d O 12 host, is proved to be reversible ( Supplementary Fig. S8 ). Even though the formation of Na6Li phase leads to a lattice volume expansion of 12.5%, we found that the excellent performance in terms of cyclic property and coulombic efficiency was achieved with the appropriate binder. This may also be rationalized by the fact that the macroscopic volume expansion is only half of the volume expansion of Na6Li lattice, namely 6.3%, as the discharged product consists of Li7 and Na6Li phases with equivalent amount, which is comparable to LiFePO 4 (6.8%), making Li 4 Ti 5 O 12 viable for reversible sodium storage. Although DFT calculations show that the Na + ion diffusion kinetics in spinel [LiTi 5 ] 16 d O 12 host is slow (note that this is not always the situation, a much better Na + ion diffusion kinetics in other structures, for example, layered Na x MO 2 (ref. 6 ), β-Al 2 O 3 (ref. 47 ), NASICON (refs 7 , 48 ), has been demonstrated. ), our full cell exhibits a moderate rate performance. This can be attributed to the shorter diffusion length and large electrode–electrolyte contact area of the used Li 4 Ti 5 O 12 nano-particles. It is generally believed that the Na + ions are too large to fit in a tetrahedral site of spinel host, and therefore the spinel type electrode for sodium-ion batteries are rarely investigated (refs 6 , 20 ), although we have demonstrated here for the first time that it is possible that the Na + ions can be reversibly introduced into the octahedral sites of the spinel host (specifically refers to [Ti 5 Li] 16 d O 12 in this case) at room temperature. This finding will provide new perspectives in the search of appropriate electrode materials for room-temperature sodium-ion batteries. Furthermore, for the insertion electrode materials in lithium- or sodium-ion batteries, a solid solution reaction (for example, layered LiNi 1/3 Co 1/3 Mn 1/3 O 2 ) or two-phase separation reaction (for example, olivine LiFePO 4 ) is always expected. However, to the best of our knowledge, this new three-phase separation mechanism of sodium storage in Li 4 Ti 5 O 12 has never been seen in the existing insertion electrode materials. Therefore, in addition to the promising applications of this new sodium storage anode material, our findings also enrich the insertion chemistry of electrode reaction and provide new perspective in understanding the electrochemical process in a battery system. Moreover, the obtained result is undoubtedly helpful in understanding the Li storage mechanism in Li 4 Ti 5 O 12 . Sample preparation The porous Li 4 Ti 5 O 12 sample was prepared by using a spray drying method as reported elsewhere [49] . The particle size was of several micrometres with about 50 nm-sized grain agglomeration together. The salt Na[N(SO 2 F) 2 ] (NaFSI) was used as received and the solvents of ethylene carbonate (EC) and diethyl carbonate (DEC) were purchased from the company of Guo Tai Hua Rong (China). The used electrolyte was 1 M NaFSI in EC:DEC (4:6 in volume). All the electrolytes were used until the water concentration was below 10 p.p.m. by removing water using the molecular sieve. Electrochemical measurements The working electrode was prepared by spreading the slurry of the active materials (80 wt.%), acetylene black (10 wt.%) and binder (10 wt.%) on Cu foil. For the PVdF binder, the solvent was N-methyl-2-pyrrolidone (NMP) for the NaAlg and Na-CMC binder, the distilled water was used as the solvent. The electrode was dried at 100 °C in vacuum for 10 h before use. The Swagelok-type cells were assembled with pure sodium foil as the counter electrode, and a glass fibre as the separator in an argon-filled glove box. The discharge/charge measurements were carried out on a Land BT2000 battery test system (Wuhan, China) at a current rate of C/10 under room temperature (C/10 refers to three Na insertion into Li 4 Ti 5 O 12 per formula unit in 10 h). The GITT experiment was performed between 3.0–0.5 V for lithium titanate electrode in the initial cycle by applying a current corresponding to a C/10 in intervals of 30 min, separated by a rest period of 12 h. Construction of a sodium-ion full cell A sodium-ion full cell was constructed using Li 4 Ti 5 O 12 as the anode and Na 3 V 2 (PO 4 ) 3 /C as the cathode in a 2032 coin-type cell. The Li 4 Ti 5 O 12 anode was prepared as shown in the above part, and the Na 3 V 2 (PO 4 ) 3 /C cathode was prepared according to our previous report [18] . The full cell was limited by the anode, in which the weight ratio (anode/cathode) of the two electrodes was 1:1.78. The electrolyte solution was 1 M NaFSI in EC:DEC (4:6 in volume). The full cells were charged and discharged between the voltage range of 1.5–3.0 V at various C-rates (C/10 current rate corresponds to 17.5 mA g −1 ). Supplementary Fig. S9 shows the first charge/discharge profile of the full cell at a current rate of C/10. Chemical sodiation The Li 4 Ti 5 O 12 powder (ca. 50 nm) was chemically sodiated by chemical reduction with sodium-biphenyl-1,2-dimethoxyethane (DME) solution as sodiating reagent. In a typical process, 87 mg pure sodium was dissolved into 10 ml colourless 1 M biphenyl-DME solution, forming a dark-green organic solution as the sodiating reagent. Then, 573 mg Li 4 Ti 5 O 12 powder was immersed into this solution (corresponding to 6 mol Na per 2 mol Li 4 Ti 5 O 12 ) and stirred until the colour of the solution fade completely to obtain the sodiated products. The products were washed by DME several times, and dried in the vacuum for overnight. The final sample was covered by the 3511 Kapton film and sealed by 502 glue for the XRD measurement. All the operations were carefully performed in the Ar-filled glove box. The sodiated product was also analysed by using the inductively coupled plasma (ICP). The ICP result indicates the molar ratio between Li and Na is 1.33, which is close to a molar ratio of 1:1 between Li7 and Na6Li phases. XRD refinement was performed with the Rietveld method as implemented in the FullProf software suite [50] and the results show a ratio of 55.5:44.5 between Li4/Li7 and Na6Li phases. This discrepancy might be attributed to the fact that the XRD measurement as a diffraction technique could only detect the Na6Li phase reaching a certain nucleus size. ICP experiments To check whether Li would be removed from Li 4 Ti 5 O 12 during the charge process, we carried out the ICP analysis on the electrolyte and the counter electrode from half cells after the cycling. The electrolyte and the passivated film on the sodium foil surface were taken from the half cell for the Li 4 Ti 5 O 12 electrode at both the charged and discharged state after 10 cycles. Then, the electrolyte and the passivated film scraped from the sodium foil surface were dissolved in water for ICP measurements. Results show that no Li could be detected in either electrolyte or the passivated film on sodium foil, indicating that the Li in the discharge product of Na 6 LiTi 5 O 12 and Li 7 Ti 5 O 12 was neither released into the electrolyte nor deposited on the counter electrode of sodium foil during the charge process. DFT calculations Spin-polarized calculations were performed using the Vienna Ab Initio Simulation Package [51] , [52] within the projector augmented-wave approach [53] . Generalized gradient approximation in the parameterization of Perdew, Burke, and Ernzerhof [54] was used to describe the exchange–correlation potential. The cutoff of the kinetic energy was set to 600 eV for all calculations. Geometry optimization was performed using a 1 a × 3 b × 1 c supercell and considered converged when the force on each atom was <1 meV A° −1 . In the model construction of Li 7− x Na x Ti 5 O 12 , different Li–Na distributions were considered. Activation barrier calculations were performed with the climbing-image nudged elastic band method [55] in a large 2 a × 3 b × 2 c supercell to minimize the interaction between the periodic images. The Brillouin zone integration was performed with 3 × 1 × 3 and 1 × 1 × 1 Γ-centred Monkhorst-Pack k-point meshes in geometry optimization and climbing-image nudged elastic band calculations, respectively. STEM imaging STEM was performed using a JEOL 2100F (JEOL, Tokyo, Japan) transmission electron microscope operated at 200 keV. The microscope was equipped with a CEOS (CEOS, Heidelberg, Germany) probe aberration corrector. The attainable spatial resolution of the microscope is 90 pm at the incident semiangle of 20 mrad. To observe Li directly using ABF collection geometry, the acceptance semiangle in this study was fixed between 10 and 20 mrad. The simulated STEM images were performed with uniform parameters, which include an accelerating voltage of 200 keV, beam direction along [110] with the specimen thickness of 50 nm (actually, the simulation with thickness range from 30 to 60 nm exhibits no qualitative difference), incident semiangle of 20 mrad, acceptance semiangle of 10–20 mrad, Cs value of 0.01 mm and a defocus of −2 nm. The image simulation was performed based on an fast-Fourier-transform multislice approach for the STEM configuration; explicit algorithm was described in detail in [56] . EDX-STEM mapping EDX-STEM mapping was performed for the Li 4 Ti 5 O 12 electrodes at both discharged and charged states in the initial cycle by a Tecnai F20 filed emission transmission electron microscope operated at 200 keV. The Ti-K, Na-K and O-K edges were used to collect chemical information of individual elements. In situ synchrotron XRD The in situ synchrotron XRD data for sodium storage into Li 4 Ti 5 O 12 were collected at Beamline BL148 ( λ =0.12398, nm) of the Shanghai Synchrotron Radiation Facility, using an image plate detector in the transmission mode. Mylar film was used as window to allow the penetration of synchrotron beam in the present in situ cell. The cell was assembled with Li 4 Ti 5 O 12 electrode as the working electrode, sodium plate as the counter electrode, 1 M NaFSI/EC:DEC as the electrolyte and Walkman glass fibre as the separator in an argon-filled glove box. The discharge/charge of in situ cell was carried on a Land BT2000 battery test system (Wuhan, China) in a voltage range of 0.5–3.0 V at a current rate of C/10. How to cite this article: Sun, Y. et al . Direct Atomic-scale confirmation of three-phase storage mechanism in Li 4 Ti 5 O 12 Anodes for room-temperature sodium-ion batteries. Nat. Commun. 4:1870 doi: 10.1038/ncomms2878 (2013).